Structural analysis of atovaquone-inhibited cytochromebc1complex reveals the molecular basis of antimalarial drug action Atovaquone, a substituted hydroxynaphthoquinone, is a potent antimalarial drug that acts by inhibiting the parasite’s mitochondrial cytochrome bc 1 complex (cyt bc 1 ). Mutations in cyt bc 1 confer atovaquone resistance. Here we describe the X-ray structure of mitochondrial cyt bc 1 from Saccharomyces cerevisiae with atovaquone bound in the catalytic Qo site, at 3.0-Å resolution. A polarized H-bond to His181 of the Rieske protein in cyt bc 1 traps the ionized hydroxyl group of the drug. Side chains of highly conserved cytochrome b residues establish multiple non-polar interactions with the napththoquinone group, whereas less-conserved residues are in contact with atovaquone’s cyclohexyl–chlorophenyl tail. Our structural analysis reveals the molecular basis of atovaquone’s broad target spectrum, species-specific efficacies and acquired resistances, and may aid drug development to control the spread of resistant parasites. Malaria is a devastating tropical disease with severe global social and economic impact. Approximately 660,000 deaths, most of them in Africa and among children, and more than 200 million cases of malaria were reported for 2010 (ref. 1 ). The infectious disease is caused by Plasmodium species, the most prevalent Plasmodium falciparum. The apicomplexan parasites are transmitted through the bites of infected mosquitoes. With a limited number of antimalarial drugs available, the emergence of acquired resistances threatens the health of individual patients as well as eradication strategies for the disease [2] . Atovaquone is a major drug used in fixed-dose combination with proguanil for treatment of uncomplicated malaria in adults and children [3] , for medicinal malaria prophylaxis [4] , and as alternative therapy in case of resistances against chloroquine or artemisin-based therapies [5] . Applications for atovaquone benefit from its broad anti-parasitic spectrum [6] . It is effectively used to treat toxoplasmosis, which is caused by the apicomplexan parasite Toxoplasma gondii , and even for pneumonia induced by the opportunistic pathogenic fungus Pneumocystis jirovecii [7] , [8] , [9] . The mode of action of the substituted hydroxynaphthoquinone atovaquone (2-[ trans -4-(4-chlorophenyl)cyclohexyl]-3-hydroxy-1,4-naphthoquinone) is based on the inhibition of mitochondrial cytochrome bc 1 complex (cyt bc 1 ; ubiquinol–cytochrome c oxidoreductase, E.C. 1.10.2.2) [10] , which is a central component of the respiratory chain and thus of cellular energy conversion [11] . As a consequence, atovaquone collapses the mitochondrial membrane potential and blocks energy supply of the parasites [12] , [13] , [14] , [15] . The drug may also act via blocking the essential pyrimidine biosynthesis, as a recent study indicates that the main metabolic function of cyt bc 1 activity in Plasmodium falciparum appears to be the regeneration of ubiquinone, which is the substrate of dihydroorotate dehydrogenase, the essential enzyme for this biosynthetic pathway [6] , [13] . The membrane-embedded cyt bc 1 couples the electron transfer from ubiquinol to cytochrome c with the vectorial translocation of protons across the lipid bilayer, thereby substantially contributing to the proton motive force that fuels synthesis of the universal energy currency adenosine triphosphate. Mitochondrial cyt bc 1 is a structural and functional homodimer with a mass of ~460 kDa consisting of 10 to 11 subunits per monomer. The catalytic core of all cyt bc 1 complexes comprises three redox-active subunits, cytochrome b (cyt b ) with two b -type haems, cytochrome c 1 (cyt c 1 ) with a c -type haem and the Rieske protein with a [2Fe-2S] cluster [11] . Cyt b is mitochondrially encoded with substantial degree of sequence and structural conservation as shown by X-ray structures of bovine, avian and yeast cyt bc 1 (refs 11 , 16 , 17 , 18 , 19 ). The enzyme mechanism, the proton motive Q cycle [20] , [21] , [22] , facilitates proton translocation by two spatially separated catalytic sites, Qo and Qi site, which are embedded in cyt b at opposite sides of the membrane. Bifurcated electron transfer on ubiquinol oxidation at the Qo site couples reduction of cytochrome c through the high potential chain and release of protons to the positive membrane side, with reduction of quinone at the Qi site and concomitant proton uptake at the opposite membrane side. The route through the high potential chain requires a conformational change of the Rieske catalytic domain, which is reduced by ubiquinol oxidation when docked onto cyt b (the b position) passing the electron to cyt c 1 after a domain movement towards the latter. The Rieske protein can be trapped in b position by Qo site inhibitors that bind the Rieske protein through the opening of the active site at the Rieske protein–cyt b interface [17] , [23] . These inhibitors bind distant to haem b L at the tip of the extended Qo site with the lipophilic tail oriented towards the ubiquinone exchange cavity, a cleft in the hydrophobic core of the enzyme at the dimer interface, which is the passage for lipophilic substrate and inhibitor molecules between the binding site and the phospholipid bilayer [16] , [24] . Atovaquone is a competitive Qo site-specific inhibitor [10] , [25] . A binding position in the active site close to the Rieske protein was suggested as the inhibitor raises the midpoint potential of the Rieske [2Fe2S] cluster by 100 mV (ref. 25 ). Atovaquone inhibits P. falciparum cyt bc 1 with high affinity in nanomolar range [26] . Similar potencies are described for other parasitic and fungal targets, but the drug also inhibits human cyt bc 1 , although with lower submicromolar affinity [27] . The molecular basis for broad target spectrum on one hand and species-specific efficacies on the other was addressed with several molecular modelling studies [25] , [28] , [29] , [30] , [31] and genetic approaches [29] , [32] , [33] , [34] , [35] , but was not resolved so far. Characterization of the binding mode is also essential to understand mutation-induced resistance. Soon after the drug was in use initially in monotherapy, mutations of parasitic cyt b arose in infected patients, above all the Y268S mutation in P. falciparum , which leads to ~9,000-fold increase in IC 50 (ref. 33 ). Mutational studies support the causal connection between mutation and resistance [30] , [35] . Yet, structural data for binding mode and molecular basis of resistance are lacking. The inherent threat of resistance requires the costly combination with proguanil, but atovaquone is very effective as combined drug [14] and accounts for instance for the majority of all pre-travel prescription in the United States [31] . Here we use mitochondrial cyt bc 1 from S. cerevisiae to elucidate the binding mode of the antimalarial drug atovaquone by means of spectroscopy, X-ray crystallography and comprehensive cyt b sequence analysis. The substituted hydroxynaphthoquinone is bound in the ionized form in the Qo site with contact to the Rieske protein. Multiple interactions with side chains of highly conserved amino acid residues dominate the binding of the napththoquinone head group. The structure sheds light on the molecular basis of broad target spectrum, species-specific efficacies, as well as acquired resistances, and may aid future drug development to control the spread of drug-resistant parasites. Crystallization of atovaquone-inhibited mitochondrial cyt bc 1 Mitochondrial cyt bc 1 from S. cerevisiae has been extensively used as a model for the highly homologous complexes from P. falciparum and other pathogens that are targeted by atovaquone [25] , [29] , [34] , [36] . The latter is a potent inhibitor of the yeast complex [25] . The enzyme activity of purified yeast cyt bc 1 is effectively inhibited by low doses of atovaquone ( Fig. 1 ). Although cyt bc 1 is a complex homodimeric enzyme in which each monomer requires three substrates, namely ubiquinol, ubiquinone and cyt c , to operate the Q cycle, dose–response titrations permit an estimate of IC 50 values for atovaquone inhibition ( Fig. 2a,b ). An extinction coefficient of ε 253 =27.3 mM −1 cm −1 for atovaquone was determined for the quantification. At pH 7.4, a pH value optimal for enzyme activity [28] , an IC 50 value of 45 nM was obtained, which agrees well with previously published data [25] . As hydroxynaphthoquinones ionize [37] and pH-dependent potency of inhibition has been reported for another ionizable cyt bc 1 inhibitor, 5-n-heptyl-6-hydroxy-4,7-dioxobenzothiazole [38] (HDBT), potency of atovaquone inhibition was monitored for a pH range between 6.5 and 7.4. In this pH range, the uninhibited enzyme activity is within ~80% of the maximum turnover [28] . With an IC 50 value of 50 nM, the potency remains high at pH 6.5 and pH 6.9 ( Fig. 1 ). The respective K i values of 2.7 nM (pH 7.4) and 3.0 nM (pH 6.5 and 6.9) are indicative for the high affinity of the inhibitor. 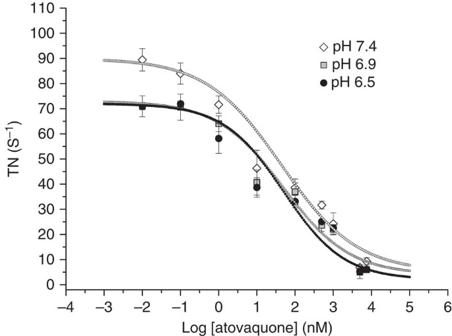Figure 1: Enzyme activity of purified yeast cytbc1is effectively inhibited by atovaquone irrespective of pH. The pH-dependent potency of inhibition was monitored by determining ubiquinol–cytochromecreductase activity (shown as turnover number (TN)) with increasing concentration of atovaquone at pH values of 6.5, 6.9 and 7.4. Dose–response curves were fitted to data points, which were measured in triplicates and are shown as average values with s.d. Figure 1: Enzyme activity of purified yeast cyt bc 1 is effectively inhibited by atovaquone irrespective of pH. The pH-dependent potency of inhibition was monitored by determining ubiquinol–cytochrome c reductase activity (shown as turnover number (TN)) with increasing concentration of atovaquone at pH values of 6.5, 6.9 and 7.4. Dose–response curves were fitted to data points, which were measured in triplicates and are shown as average values with s.d. 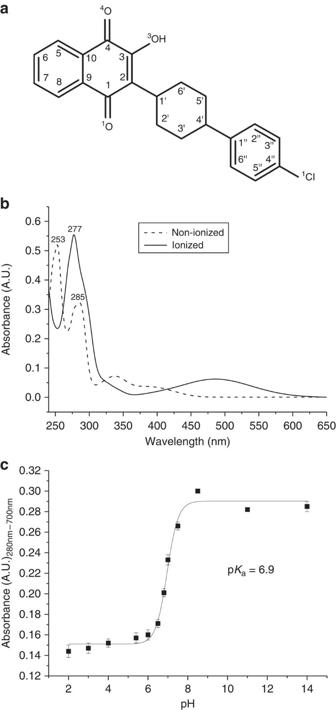Figure 2: Physico-chemical features of atovaquone. (a) Chemical structure of atovaquone (2-[trans-4-(4-chlorophenyl)cyclohexyl]-3-hydroxy-1,4-naphthoquinone). The hydroxyl group can ionize. (b) Ultaviolet–visible spectra of ionized (0.4 M KOH) and non-ionized (9% HCl) atovaquone. Characteristic for the former is an absorption maximum at 277 nm. The latter shows absorption maxima at 253 nm and 285 nm. (c) A pKaof 6.9 was determined for atovaquone in detergent solution. The absorption of atovaquone at different pH values was measured at 280 nm, at which the difference in absorption between ionized and non-ionized form is highest. The measurement was performed in eight duplicates. Average values with s.d. as well as the sigmoidal function fitted to the data points are shown. Full size image Figure 2: Physico-chemical features of atovaquone. ( a ) Chemical structure of atovaquone (2-[ trans -4-(4-chlorophenyl)cyclohexyl]-3-hydroxy-1,4-naphthoquinone). The hydroxyl group can ionize. ( b ) Ultaviolet–visible spectra of ionized (0.4 M KOH) and non-ionized (9% HCl) atovaquone. Characteristic for the former is an absorption maximum at 277 nm. The latter shows absorption maxima at 253 nm and 285 nm. ( c ) A p K a of 6.9 was determined for atovaquone in detergent solution. The absorption of atovaquone at different pH values was measured at 280 nm, at which the difference in absorption between ionized and non-ionized form is highest. The measurement was performed in eight duplicates. Average values with s.d. as well as the sigmoidal function fitted to the data points are shown. Full size image Ionized and non-ionized form of hydroxynaphthoquinones show distinct ultraviolet/visible spectra [37] , which include for atovaquone a prominent absorption maximum at 277 nm on ionization and maxima at 253 and 285 nm for the non-ionized form ( Fig. 2b ). A p K a of 6.9 was determined by spectroscopy for atovaquone in detergent solution ( Fig. 2c ). As the differences of the IC 50 values above and below the p K a are small, it indicates that the binding of the inhibitor is not influenced by its ionization state in solution. Thus, a wide pH range was kept for searching the optimal crystallization conditions. Atovaquone-inhibited yeast cyt bc 1 was crystallized with bound antibody Fv fragments. The strategy of antibody-mediated crystallization has previously been successfully used to obtain X-ray structures of the yeast enzyme with bound inhibitors and substrates [16] , [24] , [39] , [40] . The antibody binds to the Rieske protein subunit, enlarging the hydrophilic surface and mediating contacts between neighbouring molecules in the crystal lattice. Crystallization conditions were identified by extensive grid screening based on previously used compositions [16] , [24] . Best crystals were obtained at pH values at and closely below the p K a determined. Crystals were very fragile and numerous crystals were screened and analysed for final structure determination. Atovaquone is bound to cyt bc 1 in ionized form To evaluate the ionization state of atovaquone in the bound state, binding of the ligand to cyt bc 1 was monitored by difference spectroscopy at pH values above, below and at the p K a titrating the ligand from sub- to superstoichiometric concentrations ( Fig. 3 ). At substoichiometric concentrations that are at least tenfold above the IC 50 , predominant binding of atovaquone can be assumed. At pH 6.8 ( Fig. 3a ), the pH value of the crystallization condition, the spectral characteristics at substoichiometric concentrations with little or no absorption at 253 nm and an absorption maximum at ~277 nm exclude that atovaquone is bound in the non-ionized form, for which the maximum at 253 nm should be pronounced and higher than the one at ~280 nm (for comparison see Fig. 2b ). The lack of absorption at 253 nm indicates the presence of the ionized form. Increasing the concentration of atovaquone, the spectrum is dominated by the mixture of ionized and non-ionized form of the inhibitor in solution, with nearly equal absorption values at 253 and 281 nm, the latter contributed by the absorption maxima of ionized (277 nm) and non-ionized (285 nm) form. Next, binding was analysed at pH 5.8, at which 92% of atovaquone is non-ionized in detergent solution ( Fig. 3b ). Difference spectra with superstoichiometric concentrations of atovaquone show spectral characteristics of the non-ionized form with maxima at 253 and 285 nm. However, at substoichiometric concentration of the ligand, the spectra are identical with that at pH 6.8, clearly indicating that atovaquone is bound in ionized form, irrespective of environmental pH and abundance of ionized molecules present. As a control, atovaquone binding was monitored at pH 8.0 ( Fig. 3c ). Here the ionized form is reflected in the difference spectra in both, sub- and superstoichiometric concentrations of the ligand. 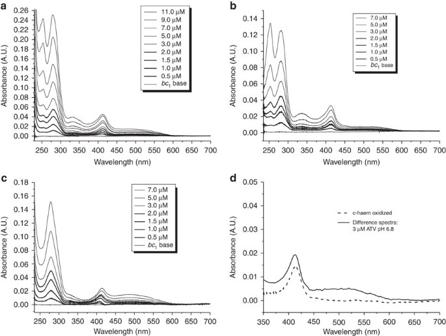Figure 3: Ionization state of atovaquone bound to cytbc1determined by difference spectroscopy. Increasing concentrations of ligand as indicated in the legend were titrated to a defined cytbc1concentration (2.1 μM). Difference spectra were recorded precisely in a dual beam set-up at (a) pH 6.8, the crystallization condition, (b) pH 5.8, at which 92% of atovaquone in solution is non-ionized and (c) pH 8.0, at which 92% of atovaquone in solution is ionized. Spectra of substoichiometric concentrations of atovaquone are highlighted in bold lines. (d) The maximum at 413 nm in the difference spectra corresponds to haem oxidation of subunit cytc1of cytbc1. The difference spectrum of potassium ferricyanide-oxidized cytbc1(dashed line) is plotted for direct comparison with an atovaquone-induced difference spectrum (solid line, 3 μM atovaquone (ATV) at pH 6.8) taken fromb. Figure 3: Ionization state of atovaquone bound to cyt bc 1 determined by difference spectroscopy. Increasing concentrations of ligand as indicated in the legend were titrated to a defined cyt bc 1 concentration (2.1 μM). Difference spectra were recorded precisely in a dual beam set-up at ( a ) pH 6.8, the crystallization condition, ( b ) pH 5.8, at which 92% of atovaquone in solution is non-ionized and ( c ) pH 8.0, at which 92% of atovaquone in solution is ionized. Spectra of substoichiometric concentrations of atovaquone are highlighted in bold lines. ( d ) The maximum at 413 nm in the difference spectra corresponds to haem oxidation of subunit cyt c 1 of cyt bc 1 . The difference spectrum of potassium ferricyanide-oxidized cyt bc 1 (dashed line) is plotted for direct comparison with an atovaquone-induced difference spectrum (solid line, 3 μM atovaquone (ATV) at pH 6.8) taken from b . Full size image All of the difference spectra feature a broad absorption maximum at ~413 nm ( Fig. 3 ). The height of the latter correlates with ligand concentration, but is not a spectral characteristic of atovaquone alone ( Fig. 2b ). Indeed, this contribution can be assigned to the oxidation of subunit cyt c 1 , as shown by comparison with a redox spectrum of cyt bc 1 alone, in which cyt c 1 is oxidized with potassium ferricyanide ( Fig. 3d ). The spectrum agrees well with the absorption spectrum of oxidized soluble cyt c [41] . The data indicate that the binding of atovaquone results in oxidation of cyt c 1 . It was described that binding of atovaquone to yeast cyt bc 1 raises the redox midpoint potential of the Rieske protein from 285 to 385 mV (ref. 25 ). The elevated potential will consequently influence the equilibration of electrons in the high potential chain. The Rieske protein that is partially reduced in the isolated enzyme [24] will withdraw electrons from cyt c 1 , which has a midpoint potential of 270 mV (ref. 42 ), thus explaining the spectrally resolved atovaquone-induced oxidation of cyt c 1 . Atovaquone binding at the Qo site of cyt bc 1 The structure of yeast cyt bc 1 with bound atovaquone was determined at 3-Å resolution ( Table 1 ). The position of the ligand in the Qo-binding site could be unambiguously assigned by its difference electron density map before including the ligand ( Fig. 4 ). The orientation of the hydroxynaphthoquinone head group is defined by the asymmetric shape of the density. The latter was well defined for the full length of the chlorophenyl–cyclohexyl tail moiety and the global-minimum conformation of the cyclohexane ring, the chair conformation, provided the best fit. The ligand was introduced in energy-minimized conformation and refined. Table 1 Data collection and refinement statistics. 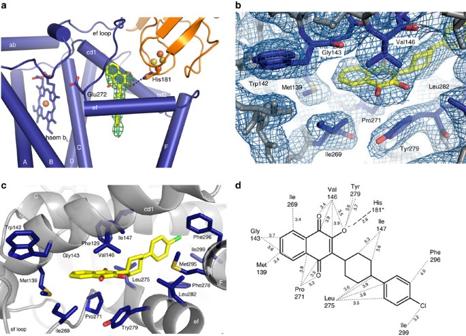Figure 4: Atovaquone binding to cytbc1. (a) View of the Qo site of the X-ray structure of yeast cytbc1with atovaquone bound. The cluster-bearing tip of the Rieske protein (orange) is docked onto cytb(blue). The polarized H-bond between the ionized hydroxyl group of atovaquone (dotted line) and the side chain of the iron–sulphur cluster ligand His181 traps the Rieske protein in thisb-position. The difference electron density map (Fo−Fc, green, contoured at 3σ) was calculated before inclusion of the ligand to the model. Transmembrane helices of cytb(tube representation) are labelled with capital letters, others in small letters. Helices G and H are removed for clarity. Cofactors and atovaquone (yellow) are shown in ball-and-stick representation. For detailed depictions, atoms are colour coded throughout the figures as indicated: oxygen, red; nitrogen, blue; chloride, cyan; iron, orange; sulphur, yellow. (b) Detailed view of the binding pocket showing head group of the inhibitor and surrounding residues of cytbwith the 2Fo−Fcelectron density map contoured at 1σ. Side chains of cytbare shown in stick representation and residues in contact with the inhibitor are highlighted in blue. The pocket is viewed from the Rieske protein, which was removed for clarity. The removal results in cutting of the density for the Tyr279 side chain, as it is in direct contact with Cys180 of the Rieske protein. (c) View of the binding site with all side chains of cytbresidues shown which contribute to atovaquone binding. The Rieske protein was removed as inb. (d) Schematic presentation of binding interactions between atovaquone and cytbc1. Interatomic distances of <4.0 Å and all contacts to the ionized hydroxyl oxygen atom are indicated in dotted lines with distances given in Å. The polarized hydrogen bond to His181 of the Rieske protein is highlighted in bold. All other contacts are from cytbresidues. For clarity, in cases of multiple interactions fulfilling the distance criterion for the same atovaquone atom, only the shortest distance is shown. A complete list of interactions is provided inSupplementary Table 1. Full size table Figure 4: Atovaquone binding to cyt bc 1 . ( a ) View of the Qo site of the X-ray structure of yeast cyt bc 1 with atovaquone bound. The cluster-bearing tip of the Rieske protein (orange) is docked onto cyt b (blue). The polarized H-bond between the ionized hydroxyl group of atovaquone (dotted line) and the side chain of the iron–sulphur cluster ligand His181 traps the Rieske protein in this b -position. The difference electron density map ( F o −F c , green, contoured at 3 σ ) was calculated before inclusion of the ligand to the model. Transmembrane helices of cyt b (tube representation) are labelled with capital letters, others in small letters. Helices G and H are removed for clarity. Cofactors and atovaquone (yellow) are shown in ball-and-stick representation. For detailed depictions, atoms are colour coded throughout the figures as indicated: oxygen, red; nitrogen, blue; chloride, cyan; iron, orange; sulphur, yellow. ( b ) Detailed view of the binding pocket showing head group of the inhibitor and surrounding residues of cyt b with the 2 F o − F c electron density map contoured at 1 σ . Side chains of cyt b are shown in stick representation and residues in contact with the inhibitor are highlighted in blue. The pocket is viewed from the Rieske protein, which was removed for clarity. The removal results in cutting of the density for the Tyr279 side chain, as it is in direct contact with Cys180 of the Rieske protein. ( c ) View of the binding site with all side chains of cyt b residues shown which contribute to atovaquone binding. The Rieske protein was removed as in b . ( d ) Schematic presentation of binding interactions between atovaquone and cyt bc 1 . Interatomic distances of <4.0 Å and all contacts to the ionized hydroxyl oxygen atom are indicated in dotted lines with distances given in Å. The polarized hydrogen bond to His181 of the Rieske protein is highlighted in bold. All other contacts are from cyt b residues. For clarity, in cases of multiple interactions fulfilling the distance criterion for the same atovaquone atom, only the shortest distance is shown. A complete list of interactions is provided in Supplementary Table 1 . Full size image Atovaquone binds at the end of the extended Qo pocket of cyt bc 1 between the [2Fe-2S] cluster of the Rieske protein and haem b L of cyt b ( Fig. 4a ). The binding pocket embedded in the latter subunit is closed by the cluster-bearing tip of the Rieske protein, which is docked on in b position. This position is enforced by a polar contact between the oxygen atom (O 3 ) of the hydroxyl group of the ligand and the nitrogen atom (NE 2 ) of the His181 side chain of the Rieske protein, a cluster ligand. With a distance of 2.8 Å between oxygen and nitrogen atoms ( Fig. 4d and Supplementary Table 1 ) and θ =130°, the hydrogen bond is in good agreement with theoretical definitions of an ideal H-bond. The above described spectroscopic analysis has clearly shown that atovaquone is bound in ionized form. Thus, the H-bond is polarized with the protonated His181 as a donor. Support for the protonated state of the latter is given by atovaquone-binding-induced cyt c 1 oxidation with concomitant Rieske protein reduction and a protonated state of His181 when the Rieske protein is reduced [43] . Both carbonyl groups of the naphthoquinone head group are without direct H-bond interaction with the side chain or main chain atoms, although water-mediated H-bonds are possible. The side chain of Glu272 of cyt b , which provides H-bond stabilization for the inhibitor stigmatellin bound to the Qo site [16] , [44] , points away from atovaquone. It is oriented towards haem b L , similar as in the structure with the bound inhibitor HDBT [24] . In the latter, a water-mediated H-bond is provided by the backbone nitrogen of Glu272 to the haem b L facing carbonyl group of the quinone ring. Such a water-mediated H-bond could also contribute to atovaquone binding. The binding site of atovaquone is flanked by transmembrane helices C, D and F, and surface helices cd1 and ef of cyt b ( Fig. 4a ). The ef loop, which carries E272 of the catalytic PEWY motif, shields the site towards the aqueous intermembrane mitochondrial space. Helices C, F, cd1 and ef, as well as the ef loop, provide numerous non-polar interactions of side- and main-chain atoms in van der Waals contact distances, stabilizing the binding of both head and tail groups of the inhibitor ( Fig. 4c,d and Supplementary Table 1 ). All interacting residues are well defined in the electron density map, indicating their distinct position (section of map shown in Figs 4b and 5 ). For the head group, contacts were identified for amino acid side chains and backbone atoms of Phe129, Met139, Trp142, Gly143, Val146, Ile269, Pro271, Leu275, Tyr279 and Leu282 of cyt b . Interactions for the tail are provided by side chains of Ile147, Leu275, Phe278, Met295, Phe296 and Ile299 of cyt b . In total, 15 residues contribute to stabilizing interactions, and the head and tail moiety of atovaquone appear to be equally well bound with multiple interactions. 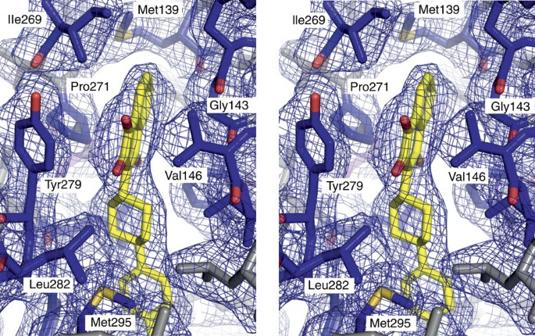Figure 5: Stereo view of the binding pocket showing the inhibitor and surrounding residues of cytochromebwith the 2Fo−Fcelectron density map contoured at 1σ. Side chains of cytbare shown in stick representation and residues in contact with the inhibitor are highlighted in blue. The pocket is viewed from the Rieske protein, which has been removed for clarity. Figure 5: Stereo view of the binding pocket showing the inhibitor and surrounding residues of cytochrome b with the 2 F o − F c electron density map contoured at 1 σ . Side chains of cyt b are shown in stick representation and residues in contact with the inhibitor are highlighted in blue. The pocket is viewed from the Rieske protein, which has been removed for clarity. Full size image A number of stabilizing contacts are of special importance for the binding, as they have multiple interactions with the ligand. These are Val146 and Gly143 of helix cd1 and Pro271, the latter a constituent of the conserved PEWY motif in the ef loop. The Val146 side chain, which is in contact to the Rieske protein, and Gly143 flank the hydroxynaphtoquinone ring plane and limit its position towards helix cd1 ( Figs 4 and 5 ). Furthermore, Tyr279 has a central role for binding ( Fig. 4b,c ). The aromatic side chain positions the hydroxynaphthoquinone ring with the two ring planes in ~59° angle while providing additional stabilization of the docked Rieske protein with a strong H-bond (2.3 Å, ϕ CZ-OH-O =120°) between its hydroxyl group and the backbone oxygen atom of Cys180. The latter is a constituent of the disulphide bond, which stabilizes the [2Fe-2S] cluster fold. The distance of δ1 and ε1 C atoms of Tyr279 and the oxygen atom of the ionized hydroxyl group is close to the sum of the van der Waals radii ( Supplementary Table 1 ); thus, the energetic contribution to ligand binding by a weak bifurcated H-bond as described for binding of ionized HDBT [24] appears to be low despite the increased acidity of the aromatic C–H groups. These differences in ligation between HDBT and atovaquone are reflected by a ~30° tilt in the ring planes of the respective head groups and correlate with a displaced position of the Rieske head group along the crystallographic y axis by 1°, as compared with HDBT [24] - or stigmatellin [39] -bound cyt bc 1 . This also highlights a certain plasticity of the active site in its closed conformation. Cyt b sequence analysis and conservation of Qo site A comprehensive analysis of amino acid residue conservation of mitochondrial cyt b was performed to evaluate the degree of conservation in the atovaquone-binding pocket. All 3,595 mitochondrial cyt b sequences were retrieved from the NCBI reference sequence mitochondrial protein database [45] . The search was based on the carboxy-terminal domain definition (PROSITE [46] ) and the corresponding profile hidden Markov model (HMM_cybC) calculated by HMMER3 (ref. 47 ). After alignment of sequences with Clustal Omega [48] and manual curation (see Methods), the complete database SEQ_cytb mito comprises 3,556 entries. To eliminate the effect of redundant sequences on diversity, homologous sequences of cyt b with identities >60% were clustered by CD-HIT [49] and the database was reduced to 130 single representative sequences ( Supplementary Table 2 ) of the clusters, to which the sequence of cyt b from S. cerevisiae was added, resulting in the comprehensive, yet non-redundant database of mitochondrial cyt b (SEQ n-r _cytb mito ). The latter information was mapped on the structure of cyt bc 1 with bound atovaquone to evaluate the degree of conservation in the binding pocket ( Fig. 6a ). 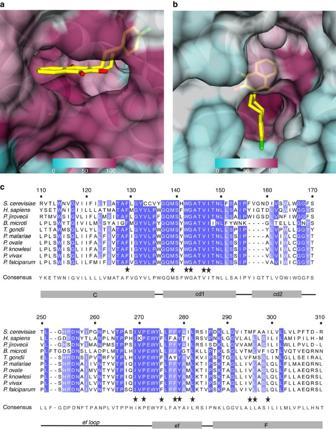Figure 6: Amino acid residue sequence conservation of the atovaquone binding pocket. (a,b) Degree of conservation was determined with the non-redundant SEQn-r_cytbmitoclustering data base and mapped on cytbshown in surface representation with bound atovaquone (yellow). The colour profile magenta to cyan covers 100 to 0% sequence conservation identity. The binding pocket is viewed inafrom the Rieske protein with the latter removed, and inbfrom the quinone exchange cavity. (c) Comparison of cytbsequences of target and model organism for atovaquone inhibition of cytbc1. Alignments for two sections of cytbsequences are shown, which cover all residues that have side-chain interactions with atovaquone in the structure. The sections are retrieved from the multiple sequence alignment of the complete SEQ_cytbmitodata base, of which the consensus sequence is shown. Dark and light blue indicate residues that show complete or up to 80% identity, respectively. Sequence numbering refers toS. cerevisiaecytb. Residues with side-chain interactions with atovaquone are labelled with a star. Secondary structural elements16,44with helices shown as grey boxes are shown at the bottom. Figure 6: Amino acid residue sequence conservation of the atovaquone binding pocket. ( a , b ) Degree of conservation was determined with the non-redundant SEQ n-r _cytb mito clustering data base and mapped on cyt b shown in surface representation with bound atovaquone (yellow). The colour profile magenta to cyan covers 100 to 0% sequence conservation identity. The binding pocket is viewed in a from the Rieske protein with the latter removed, and in b from the quinone exchange cavity. ( c ) Comparison of cyt b sequences of target and model organism for atovaquone inhibition of cyt bc 1 . Alignments for two sections of cyt b sequences are shown, which cover all residues that have side-chain interactions with atovaquone in the structure. The sections are retrieved from the multiple sequence alignment of the complete SEQ_cytb mito data base, of which the consensus sequence is shown. Dark and light blue indicate residues that show complete or up to 80% identity, respectively. Sequence numbering refers to S. cerevisiae cyt b . Residues with side-chain interactions with atovaquone are labelled with a star. Secondary structural elements [16] , [44] with helices shown as grey boxes are shown at the bottom. Full size image The terminal cavity of the binding pocket, which encloses the hydroxynaphthoquinone head group moiety of atovaquone, is lined nearly completely with highly conserved residues ( Fig. 6a ). Towards the tail region of the ligand, the surface residues of the binding pocket are less conserved ( Fig. 6b ). This end of the pocket opens up towards a hydrophobic cleft at the cyt bc 1 dimer interface, which is the passage for inhibitor and substrate molecules. In detail, amino acids interacting with the head group are located in helices C, cd1 and ef, and in the ef loop. Contacts with side-chain atoms as compared with main-chain atoms ( Supplementary Table 1 ) dominate the binding. Residues contributing side-chain interactions are with one exception fully conserved as compared with the consensus sequence of all mitochondrial cyt b sequences ( Fig. 6c ). Thus, they are also present in the atovaquone target organism analysed here with apicomplexan ( Plasmodium malariae , Plasmodium ovale , Plasmodium knowlesi , Plasmodium vivax , T. gondii , Babesia microti ) or fungal origin ( P. jirovecii ) ( Fig. 6c and Table 2 ). The only exception, Leu275, is not only present in S. cerevisiae , but also in B. microti and P. jirovecii , whereas phenylalanine harbours this position in Plasmodium strains, T. gondii and Homo sapiens , as well as in the consensus sequence. The interactions with the tail ring moieties are exclusively contributed from side chains and comprise fully conserved Ile147 ( Fig. 6c and Table 2 ) of helix cd1 and the less conserved residue Phe278 of helix ef and Met295, Phe296 and Ile299 of helix F ( Fig. 6c and Table 2 ). Phe278 is present in all apicomplexan targets except in T. gondi , in which it is replaced by tyrosine. Interestingly, alanine is at this position in the consensus sequence and is also present in H. sapiens . Residues of helix F show conservative replacements. Ile299 is also present in T. gondii , B. microti and P. jirovecci , whereas the other two residues vary among species. The comprehensive sequence alignment confirmed that the four amino acid deletion in the cd2 helix [26] is exclusively found in apicomplexa ( Fig. 6c ). The helix is positioned parallel to the cd1 helix, which flanks the active side ( Fig. 4a,c ). None of the four respective residues (Phe156, Val157, Gly158 and Asn159) is in direct contact with atovaquone; however, the side chains are oriented towards the transmembrane helix of the Rieske protein. Table 2 Degree of sequence conservation for amino acids in contact with ATV. Full size table The stabilization of the naphthoquinone head group by interactions with conserved residues supports the relevance of yeast cyt bc 1 as a model for the pathogenic complexes. In the tail region, species-specific interactions may occur as surface residues are less conserved and the tail region of atovaquone may rotate to facilitate other contacts. The structurally resolved, well-defined binding position of atovaquone in the Qo site of yeast mitochondrial cyt bc 1 fully agrees with its highly efficient, ubiquinol competitive inhibition of the enzyme. Notably, the spectroscopic analysis presented here clearly demonstrates that atovaquone is bound in its ionized form, irrespective of pH and abundance of the non-ionized form. Previously, this ionization was not taken into account and atovaquone binding was modelled in several docking studies with its non-ionized hydroxyl group interacting with His181 of the Rieske protein [25] , [28] , [29] , [30] , [50] . In general, ionization of the hydroxyl group of hydroxynaphthoquinones is known and p K a values are described in the range of 4.7–6.8 (ref. 37 ). We determined a p K a of 6.9 for atovaquone in detergent solution. The selective binding of the ionized form is in agreement with the finding that atovaquone binding raises the midpoint potential of the Rieske protein substantially [25] , thus favouring binding of the ligand to the reduced subunit. The latter is supported by the spectroscopically observed atovaquone-induced oxidation of subunit cyt c 1 , which can be explained by a re-equilibration of electrons towards the Rieske protein. Furthermore, reduction of the Rieske protein raises the p K a of His181 to above 11 as compared with ~7.5 for the oxidized form [11] , [43] . At physiological relevant pH, His 181 is protonated in the reduced Rieske protein and thus is a capable H-bond donor. The electrostatic component and delocalization of charges by equilibration of electrons strengthens the binding of the ionized hydroxyl group of atovaquone with a polarized H-bond. The polarized binding mode appears to be energetically favourable as compared with a non-ionized atovaquone molecule donating a H-bond to the non-protonated His181 of an oxidized Rieske protein. A possible higher binding affinity of atovaquone to reduced cyt bc 1 complex needs to be addressed in future studies. The binding most probably mimics the stabilization of the transition state of ubiquinol oxidation, which provides the basis for the bifurcated electron transfer involving concomitant electron and proton transfer from ubiquinol to the Rieske protein. The trans isomer of atovaquone, which is substantially more potent than the cis isomer [31] , is bound in the active site in the energetically favourable chair conformation. The hydroxynaphthoquinone head group snugly fits into the terminal cavity of the binding pocket, whereas the cyclohexyl group is stabilized in the slightly wider part of the cavity that opens towards the ubiquinone exchange cavity at the dimer interface. Interestingly, the numerous non-polar interactions between cyt b and atovaquone that stabilize binding in addition to the polarized H-bond are in large majority contributed by amino acid residue side chains ( Supplementary Table 1 ). Only 8 out of 47 interactions are provided by main-chain atoms. In addition, these residues are highly conserved among all mitochondrial cyt b sequences. The high conservation of Qo site surface residues in the terminal cavity is most likely to be driven by the requirement for precise positioning and binding of the ubiquinol substrate in the active site important for its undisturbed oxidation. For instance, the mutations Y279A and F129K in yeast substantially lower the enzyme activity to below 30% of wild-type turnover [51] . In addition, these mutations result in bypass reactions that generate deleterious reactive oxygen species. The high degree of conservation relevant for the inhibitor binding appears to be the molecular basis for the broad target species spectrum of atovaquone. The majority of the respective residues (Phe129, Met139, Trp142, Gly143, Val146, Ile147, Ile269, Pro271, Tyr279, Leu282) are identical in cyt b of yeast, malaria parasites ( P. falciparum , P. vivax , P. knowlesi , P. ovale , P. malariae ), pneumonia-causing P. jirovecii , babesiosis-causing B. microti and toxoplasmosis-causing T. gondii , as well as humans ( Fig. 6c ), and they have a very high sequence conservation for all mitochondrial cyt b ( Table 2 ). This group includes Gly143, Val146 and Pro271, which have multiple interactions with the ligand. Pro271 is constituent of the PEWY motif of ubiquinol oxidation and is 100% conserved among all cyt b sequences. In the tail region, residues can be linked to species-specific binding. Phe278 is present in all but one target organism, namely T. gondii , in which it is replaced by tyrosine. This conservative replacement may have little effect on the binding mode. Interestingly, alanine is present at this position in the consensus sequence (89% conserved, Table 2 ) as well as in man. The phenylalanine side chain is in contact with Ile299 and its alanine substitution could destabilize binding interactions to the chlorophenyl ring and consequently lower the potency of atovaquone for inhibition of human cyt bc 1 (IC 50 between 70 nM (ref. 26 ) and 460 nM (ref. 27 )) depending on the study and cell type used as compared with P. falciparum (IC 50 =3.0 nM (ref. 26 )). Even more natural diversity is seen for a ligand of the cyclohexyl ring, Leu275, which is present in S. cerevisiae and also in P. jirovecii and B. microti , whereas a phenylalanine is present at this position in Plasmodium species and T. gondii ( Fig. 6c ). The L275F mutation in yeast showed no effect on enzyme activity but a tenfold increase of the IC 50 (ref. 25 ). The residue is also of interest for mutation-induced resistances, which will be discussed below. In conclusion, the data strongly indicate that the hydroxynaphthoquinone head group binding is conserved among species, whereas specificity arises from interactions with the tail group. Initial atovaquone monotherapy gave rapid rise to resistance correlated with cyt b mutations [14] . The causal link between mutations and acquired resistance can be assessed in S. cerevisiae , as the yeast is amenable to mitochondrial transformation and mutations can be introduced for cyt b [34] . Resistances are not expected to arise for residues that are crucial for functional integrity of the enzyme. Yet, substitutions without major loss of enzyme activity can lower inhibition efficiency, either by deleting interactions or by introducing sterical hindrance. The most prevalent mutation that is associated with acquired atovaquone resistance in P. falciparum is Y268S [30] , [33] (Y279S in yeast numbering). The yeast mutation Y279S [28] , [32] , [35] showed a ~40-fold increased IC 50 (~1.7 μM) for atovaquone as compared with the wild type [35] . The structure suggests a crucial function of this residue for atovaquone binding, as the aromatic ring of the highly conserved residue (98%, Table 2 ) positions the ionized hydroxyl group, which provides the central polar contact to the Rieske protein. In addition, Y279 stabilizes the docked b position with a H-bond between its hydroxyl group and C180 of the Rieske protein. Resistance-related mutations arose also for contacts in the tail region. The mutations I147V and L275F identified in a cohort study of AIDS patients with P. jirovecii infection [52] , showed in yeast cyt bc 1 two- and eightfold increased IC 50 values, respectively [53] . Both side chains interact with the cyclohexyl ring of the tail ( Fig. 4c,d ), while the leucine side chain also has a single contact with the quinone ring of the head group. The elevated IC 50 of L275F was previously discussed as explanation for lower atovaquone sensitivity of bovine and human complexes, which naturally have the residue Phe275 (ref. 25 ). This conclusion is contradictory to the fact that Phe275 is also present in the Plasmodium species, which are highly sensitive to the drug. The L275F resistance can now be explained with the ligation of the cyclohexyl ring. The expected slight shift of the cyclohexyl ring in the presence of Phe275 as compared with that of leucine could be compensated by a matching residue on the opposite side of the ring, namely Val295 in Plasmodium targets, whereas Met295 in yeast cannot fully accommodate this shift, resulting in the elevated IC 50 . In support of this hypothesis, the Leu275-carrying P. jirovecii and B. microti also naturally harbour Met295. Taken together, there is strong evidence that the binding mode of atovaquone revealed for the mitochondrial yeast cyt bc 1 resembles in essence the interaction of the drug with the complexes of target organisms. It explains the molecular basis for the broad target spectrum of the parasitic drug as well as for the species-specific differences in efficacy. These data further the understanding of drug resistance and may enable improvement of drugs that target cyt bc 1 . Antibody-mediated crystallization of cyt bc 1 with atovaquone Complex formation of cyt bc 1 from S. cerevisiae and the antibody fragment Fv 18E11 was performed as previously described [16] . In short, proteins were produced, purified and combined at 1.2-fold molar ratio. Cyt bc 1 was quantified by redox spectroscopy of haem b L and haem b H ( ε 562–575 =28.5 mM −1 cm −1 for dithionite-reduced minus ferricyanide-oxidized cyt bc 1 difference spectra) [24] . Excess Fv fragment was subsequently removed by size exclusion chromatography. Atovaquone (A7986 Sigma, purity ≥98%), dimethylsulphoxide (DMSO) and sucrose were added to the complex (10 mM Tris, pH 8.5) before crystallization at final concentrations of 80 μM (1.3-fold molar excess), 10% and 250 mM, respectively. Crystallization conditions were identified with systematic grid screens based on previous conditions for cyt bc 1 crystals with Qo site inhibitors [16] , [24] . Final crystals were grown with vapour diffusion technique at 4 °C. Protein solution (60 mg ml −1 ) was mixed in 1:1 proportion with precipitation solution (5.5% polyethylene glycol 4,000, 150 mM KPi pH 6.8, 0.05% n-undecyl-β- D -maltopyranoside (UM), 10 μM atovaquone) and crystals grew within a few days to a suitable size (≈0.2 mm × 0.5 mm × 0.8 mm). Cryo conditions were obtained by increasing the sucrose concentration stepwise to 750 mM before flash-cooling in liquid nitrogen. Atovaquone analysis by optical spectroscopy Atovaquone stock solution (20 mM in DMSO) was diluted 1:1,000 in 99% p.a. ethanol (EtOH). Reference spectra of non-ionized and ionized form of atovaquone were measured in acidified (9% HCl) and alkaline (0.4 M KOH) EtOH with 99% EtOH as baseline. The extinction coefficient ε at 253 nm was determined gravimetricly for atovaquone in acidified 99% p.a. EtOH (20 mM HCl) as the mean value from three experiments, each with individual stock solutions and triplicate spectra. All spectra were recorded with a Cary 4000 ultraviolet–visible spectrophotometer. The p K a of atovaquone was determined in detergent containing solution buffered at different pH values. Atovaquone (20 μM) was diluted from stock solution in the following buffers supplemented with 0.5% UM: 9% HCl pH 2, 250mM citrate buffer pH 3–4, 250mM KPi pH 5.5–6.5, 250mM Hepes pH 7–7.5, 250mM Tris pH 8.5, 250mM CAPS pH 11, 0.4 M KOH pH 14. For each pH value, the absorption at 280–700 nm was determined in 8 duplicates with a ultraviolet-transparent 96-well plate (UV-star microplate, Greiner Bio-one) in a plate reader (BioTek Power Wave XS2) and mean value±s.d. was calculated. Values were plotted with Origin Pro 8.1, a sigmoidal function (Boltzmann model) was fitted and the inflection point (x0) determined. Determination of the protonation state of bound atovaquone Difference spectra of cyt bc 1 and cyt bc 1 with increasing concentrations of atovaquone were recorded in double beam configuration with Z20 cuvettes (10 mm, Starna Scientific Ltd) at the Cary 4000 ultraviolet–visible spectrophotometer. Cyt bc 1 (2.1 μM) in buffered solution (0.05% UM, 0.5 M sucrose, 150 mM citrate buffer pH 5.8 or KPi buffer pH 6.8) was used for the reference cuvette. In the other cuvette, the same sample was titrated with atovaquone from substoichiometric to superstoichiometric amounts (0.5, 1, 1.5, 2, 3, 5, 7, 9, 11 μM). For analysis of cytochrome c 1 oxidation, a difference spectrum of oxidized cyt bc 1 (12 μM potassium ferricyanide (K 3 [Fe(CN) 6 ])) minus cyt bc 1 as isolated was measured in dual beam mode and the spectrum of potassium ferricyanide alone was subtracted. Plots of the absorption spectra were generated in OriginPro 8.1. IC 50 determination for atovaquone inhibition of cyt bc 1 Ubiquinol:cytochrome c reductase activity was determined at varying concentration of atovaquone at different pH values. Reaction volumes of 1 ml contain 5 nM cyt bc 1 , 16 μM horse heart cytochrome c and 100 μM ubiquinol in the respective assay buffer (50 mM KPi pH 6.5, 6.9, and 7.4 with 0.2 mM EDTA, 1 mM NaN 3 , 250 mM sucrose, 0.05% UM). The reaction was started with ubiquinol. Reduction of cyt c was monitored at 550 nm for 1 min and the initial linear rate quantified ( ε =19 mM −1 cm −1 ). Measurements were performed at different final inhibitor concentration in the range of 0.01 nM to 7.5 μM ( ε 253 =27.3 mM −1 cm −1 ) with a constant final DMSO concentration of 0.02%. Dose–response curves were fitted with Origin Pro 8.1 to data points, which were measured in triplicates (±s.d.) and IC 50 values calculated from the dose–response fits with the following formula: fixing A1 and A2 and fitting x0 (IC 50 ), and p. K i values were calculated as described before [25] using the determined IC 50 values and the following formula with the previously determined K M of 6.3 μM (ref. 51 ). Data collection, structure determination and refinement X-ray diffraction data were collected at 100 K at the synchrotron beamline PXIII at the Swiss Light Source (Paul-Scherrer-Institut, Villigen, Switzerland) with a wavelength of 1.0 Å and a Pilatus 2 M detector. Data were processed and scaled with the XDS programme package (version: 26 September 2012) [54] . The crystal belongs to the space group C2 with cell parameters of a =212.3 Å, b =151.0 Å, c =143.1 Å, β =115.2 ( Table 1 ). The structure was solved by molecular replacement (PHENIX v. 1.8) [55] using a monomer of the 1.9-Å resolution structure of cyt bc 1 (pdb code: 3CX5) [39] as search model. Insertion of ligands and modelling was done using the programme COOT (version 0.6.2) [56] . An energy-minimized coordinate file of atovaquone was generated using the GlycoBioChem PRODRG2 Server [57] and a geometry restraint library file was generated from the coordinates with sketcher/libcheck of the CCP4i programme package v. 6.3.0 (refs 58 , 59 ). Few amino acid displacements including side chains of Qo site residues Glu272, Tyr279, Tyr132, Tyr 136, Leu150and Met295 of cyt b were manually adjusted, followed by stepwise inclusion of the energy-minimized structures of phospholipids, ubiquinone-6, UM and atovaquone. In addition, the peptide bonds of His222/Ser223 and Val346/Pro347 of cyt b were changed to cis conformation. Each step of model building was followed by a refinement cycle with restrained, individual B factor and occupancy refinement using phenix.refine. Ramachandran analysis by Molprobity showed 80.8% and 15.5% for favoured and allowed regions, respectively, and 3.7% for outliers. Sequence alignment and amino acid conservation of cyt b For comprehensive sequence analysis, cytochrome b protein sequences were identified by their C-terminal domain, which is defined in the PROSITE database [46] . Representative sequences of the domain were obtained from the latter and the corresponding profile hidden Markov model (HMM_cybC) was calculated by HMMER3 (ref. 47 ). All mitochondrial cytochrome b protein sequences (3,595) were retrieved from the NCBI RefSeq database (release 59) [45] . After multiple sequence alignment of all sequences with Clustal Omega [48] , homologues were deleted, which feature gaps for the axial ligands of the two b -type haems (His82, His96, His183 and His197) or for the PEWY motif; the latter includes the putative ubiquinol ligand Glu272. Sequences that do not cover the full length of yeast cyt b and those that generate single insertions or deletions as compared with all sequences were also removed. The remaining sequences constitute the complete database SEQ_cytb mito with 3,556 entries. For the non-redundant database (SEQ n-r _cytb mito ), CD-HIT [49] was used for clustering homologous sequences from SEQ_cyt mito based on identities >60%. The database was reduced to 130 single representative sequences of the clusters ( Supplementary Table 2 ) and the sequence of cyt b from S. cerevisiae was included for comparison. All the aforementioned programmes were standalone releases and were executed with default settings and parameters. The graphical output of the sequence alignment was generated with the programme Jalview 2.8 using the percentage identity function. Secondary structural elements were added with Corel Draw X5. The programme Chimera [60] was used to map the degree of cyt b sequence conservation on the cyt bc 1 structure for evaluation of the atovaquone binding site. Degree of conservation is based on multiple sequence alignment [48] of the non-redundant database SEQ n-r _cytb mito . In the Render/select by Attribute function, mavPercentConserved was chosen as the attribute to colour the amino acid residues according to their conservation. Accession codes: Coordinates and structure factors of the structure were deposited in the RCSB Protein Data Bank under accession code 4PD4 . How to cite this article: Birth, D. et al. Structural analysis of atovaquone-inhibited cytochrome bc 1 complex reveals the molecular basis of antimalarial drug action. Nat. Commun. 5:4029 doi: 10.1038/ncomms5029 (2014).